RETRACTED ARTICLE: Mir20a/106a-WTX axis regulates RhoGDIa/CDC42 signaling and colon cancer progression Wilms tumor gene on the X chromosome ( WTX ) is a putative tumor suppressor gene in Wilms tumor, but its expression and functions in other tumors are unclear. Colorectal cancer (CRC) is the third leading cause of cancer-related deaths in women and the second leading cause in men in the United States. We demonstrated that WTX frequently lost in CRC which was highly correlated with cell proliferation, tumor invasion and metastasis. Mechanistically, WTX loss disrupts the interaction between RhoGDIα and CDC42 by losing of the binding with RhoGDIα and triggers the activation of CDC42 and its downstream cascades, which promotes CRC development and liver metastasis. The aberrant upregulation of miR-20a/miR-106a were identified as the reason of WTX loss in CRC both in vivo and in vitro. These study defined the mechanism how miR-20a/miR-106a-mediated WTX loss regulates CRC progression and metastasis, and provided a potential therapeutic target for preventing CRC progression. WTX, also known as FAM123B or AMER1, not only is it the first tumor suppressor gene located on X chromosome, as it was identified in Wilms tumor [1] , it also plays an important role in embryonic development and organ differentiation [2] . As an important factor in Wnt/β-catenin pathway, WTX forms a complex with β-catenin, AXIN1, β-TrCP2 (beta-transducin repeat-containing protein 2), and APC (adenomatous polyposis coli). WTX promotes β-catenin ubiquitination and degradation, which antagonizes WNT/β-catenin signaling in Wilms tumor [3] . However, the expression level of WTX is unknown and the functions of WTX are not fully elucidated in other kinds of tumors. Our previous study found that WTX was commonly lost in colorectal cancer (CRC) [4] . CRC is the third leading cause of tumor-related deaths attributed to vital organ metastasis [5] . Liver metastases occur in one fourth of CRC patients, and about 70% of them died from liver metastases [6] . In this study, we discovered that loss of WTX could activate CDC42 through disrupting the interaction between CDC42 and its inhibitor Rho GDP-dissociation inhibitors (RhoGDIa), which promotes F-actin nucleation, polymerization, and further CRC liver metastasis. In addition, our study had also shown that WTX loss is highly correlated with poor prognoses of CRC patients. As a tumor suppressor gene in X chromosome, in contrast to the “double-hit” mutation system of the most autosome located tumor suppressor genes, WTX can be inactivated by a monoallelic “single-hit” mutation, which indicates that somatic WTX loss can be achieved by one “hit” on the X chromosome of males or the active X chromosome of females. The mutation was the first mechanism found to drive WTX silencing in Wilms tumor, with a mutation rate ranged for ~30% [7] or even lower rates in Wilms tumors [8] , [9] . However, the mutation driven WTX silencing is rare and diverse in hepatoblastoma and CRC patients [10] , [11] , [12] , [13] , it suggests that there might be some other mechanisms responsible for WTX gene silencing and loss in those patients. Aberrant microRNA (miRNAs) regulation is a well-known cause of target gene silencing in addition to gene mutation. MiRNAs are 19-25 nucleotides in length and can specifically bind to target genes and inhibit gene expression. They regulate at least one-third of human genes and play important roles in cell proliferation, apoptosis [14] , differentiation [15] , gene regulation [16] , and tumorigenesis [17] . In addition, miRNA dysregulation has been reported to mediate CRC development via posttranscriptional regulation of target gene expression [18] , [19] . Although upregulation of microRNA-370 has been reported to inhibit WTX expression in Wilms tumors [15] , whether WTX loss in CRC is mediated by miRNAs remains unknown. To investigate the effect of miRNAs on WTX loss and uncover the mechanism of WTX loss in CRC, we performed the miRNA expression profiling of human CRC samples with high and low WTX expression. WTX loss correlates to CRC liver metastasis and poor prognoses Previous studies by our team revealed that WTX was lost in CRC patients, but the clinical value of WTX loss was not fully evaluated [4] . To further determine the role of WTX in CRC progression and metastasis, a total of 117 cases of CRC samples and paired colorectal mucosa were collected and performed Immunohistochemistry (IHC) staining in this study. It confirmed that WTX loss has a significane higher frequency in CRC (89/117, 76.1%) than in normal tissues (17/117, 14.5%) ( p < 0.0001) (Fig. 1a ). 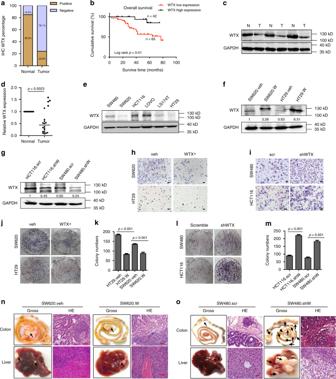Fig. 1 WTX loss promotes CRC cells, migration and liver metastasis.aPercentage of WTX IHC in CRC and matched adjacent normal colorectal mucosa tissues.bKaplan–Meier survival analysis of CRC patients with WTX high or WTX low expression.cImunoblotting (IB) analyzes the WTX expression in human CRC tumor (T) and matched adjacent normal mucosa (N) tissues.dqRT-PCR analyzes WTX mRNA level in human CRC tumor and matched adjacent normal mucosa tissues. **p= 0.0023, mean ± SEM. Two-tailed Student’st-test.eIB analyzes WTX expression in CRC cell lines.f,gIB analyzes WTX expression in indicated cell lines.h,iTranswell analyzes the migration of the indicated cell lines. Scale bars, 200 μm.j–mColony formation analysis of the indicated cell lines. ***p< 0.001, mean ± SEM. Two-tailed Student’st-test.n,oGross and H&E staining observe the CRC orthotopic tumors and liver metastasis in indicated cell lines. Each arrow pointed a tumor mass. Scale bars, 20 μm,n= 11 (n) andn= 8 (o) Also, WTX loss was higherly correlated with liver metastasis ( p = 0.0055), WHO stage classification ( p = 0.0086) and poor survival rate ( p = 0.0094) of CRC patients (Table 1 and Fig. 1b ). Immunoblotting and quantitative qRT-PCR were further implemented and verified WTX loss at both the protein (Fig. 1c ) and mRNA (Fig. 1d , p = 0.0023) levels in CRC patients. These results suggest that WTX is a potential tumor suppressor and prognostic marker in CRC patients and WTX loss may play an important role in promoting CRC progression and metastasis. Fig. 1 WTX loss promotes CRC cells, migration and liver metastasis. a Percentage of WTX IHC in CRC and matched adjacent normal colorectal mucosa tissues. b Kaplan–Meier survival analysis of CRC patients with WTX high or WTX low expression. c Imunoblotting (IB) analyzes the WTX expression in human CRC tumor (T) and matched adjacent normal mucosa (N) tissues. d qRT-PCR analyzes WTX mRNA level in human CRC tumor and matched adjacent normal mucosa tissues. ** p = 0.0023, mean ± SEM. Two-tailed Student’s t -test. e IB analyzes WTX expression in CRC cell lines. f , g IB analyzes WTX expression in indicated cell lines. h , i Transwell analyzes the migration of the indicated cell lines. Scale bars, 200 μm. j – m Colony formation analysis of the indicated cell lines. *** p < 0.001, mean ± SEM. Two-tailed Student’s t -test. n , o Gross and H&E staining observe the CRC orthotopic tumors and liver metastasis in indicated cell lines. Each arrow pointed a tumor mass. Scale bars, 20 μm, n = 11 ( n ) and n = 8 ( o ) Full size image Table 1 The correlation of WTX expression with the clinicopathological features of CRC Full size table WTX loss promotes CRC proliferation, migration, and liver metastasis To further investigate the function of WTX in CRC development, the endogenous expression of WTX was analyzed in six CRC cell lines (SW480, SW620, HCT116, Lovo, LS174T, and HT29) (Fig. 1e ). Analyze result shown a high expression of WTX in SW480, HCT116, and LOVO cell lines, in contrast, in SW620, HT29, and LS174T cell lines WTX expression was relatively low. Two stable WTX-overexpressing cell lines SW620(SW620.W), HT29(HT29.W) (Fig. 1f ) and two WTX knockdown cell lines SW480(SW480.shW) and HCT116(HCT116.shW) (Fig. 1g ) were established for the following in vitro and in vivo experiments. Cell migration (Fig. 1h and Supplementary Fig. 1a ) and colony formation ability (Fig. 1j, k ) were significantly inhibited compared with control cells (SW620.veh and HT29.veh) after WTX overexpression (SW620.W and HT29.W). In contrast, the migration (Fig. 1i and Supplementary Fig. 1b ) and colony formation (Fig. 1l, m ) ability of the cells were significantly increased compared with control cells (SW480.SCR and HCT116.SCR) after WTX knockdown (SW480.shW and HCT116.shW). The migration inhibiting function of WTX was validated by wound-healing assays (Supplementary Fig. 1c–f ). 3D culture also confirmed that SW620 cell proliferation was inhibited when WTX was overexpressed (Supplementary Fig. 1 g, h ). These set of data suggest that WTX inhibits CRC cell malignant progression and migration. To farther investigate the functions of WTX in vivo, the tumor growth of WTX high or low expressing CRC cells were observed by using the subcutaneous xenograft tumor models. It revealed that WTX can negatively regulate CRC tumor growth (Supplementary Fig. 2a–d ). The orthotropic xenograft tumor models were also established to observe the tumor growth and metastasis. The data shown that SW620.veh group exhibited 100% (11/11) colorectal tumor formation, with 63.6% (7/11) high tumor burdens and liver metastasis, and the SW620.W group showed 45.5% (5/11) colorectal tumor formation, with low tumor burden (all of the tumor mass were no more than 1 cm in diameter) and no liver metastasis (Fig. 1n , Supplementary Fig. 2e and Supplementary Table 1 ). On the other hand, the SW480.SCR group has a 62.5% (5/8) colorectal tumor formation rate, low tumor burdens, and no liver metastasis. The SW480.shW group exhibited 100% (8/8) colorectal tumor formation with high tumor burdens (100%), and 75% (6/8) of cases progressed to liver metastasis (Fig. 1o , Supplementary Fig. 2f and Supplementary Table 1 ). The in vitro and in vivo results confirm that WTX functions as a tumor metastasis suppressor gene which can dramatically inhibit CRC progression and liver metastasis. Inhibition of CDC42 prevents the WTX loss induced CRC cell migration To investigate how WTX loss promotes CRC metastasis, two-dimensional page electrophoresis (2-DGE) and mass spectrometry analysis were used to identify those altered protein expressions induced by WTX overexpression in SW620.W cells compared to SW620.veh cells. Seventy-six proteins were identified from 90 differential protein dots (DPDs) and classified according to biological function. Compared with SW620.veh cells, the regulators of cytoskeleton dynamics were dramatically changed in SW620.W cells. These differential proteins includes the cytoskeleton stabilization-promoting factors Myo1c (unconventional myosin-Ic), FMNL3 (Formin-Like 3), CAPZA1 (F-actin-capping protein subunit alpha-1), and TTLL5 (Tubulin tyrosine ligase like 5), these proteins were all downregulated following overexpression of WTX (Supplementary Fig. 3a and Fig. 2a ). This suggests that WTX might play a role in regulating the cytoskeleton protein stabilization. Fig. 2 Inhibition of CDC42 activity prevents WTX loss induced CRC cell migration. a 2-DGE searches the difference protein expression dots between SW620.veh and SW620.W cells. Scale bars, 500 μm. b CO-IP analyzes the interaction of WTX and Small GTPases family members in SW620.W cells. c IF staining analyzes the colocation of WTX and CDC42 in SW620.veh and SW620.W cells. Scale bars, 10 μm. d IB analyzes the expression level of CDC42 and CDC42 GTP in indicated cell lines. e , f IB analyzes the expressions of WTX, CDC42 and CDC42 GTP in indicated cells. g , h Transwell experiments analyze the migration ability in indicated cells. Scale bars, 200 μm. i , j IHC staining analyzes the expressions of CDC42 and CDC42 GTP in CRC orthotopic tumors. Scale bars, 20 μm Full size image Rho family small GTPase members are important regulators of cell migration through mediating cytoskeleton stabilization [20] , [21] . We hypothesized that WTX might regulate cytoskeleton stabilization through Rho family small GTPase members. There are three known small GTPase members, RhoA, RAC1, and CDC42 (Cell Division Cycle-42) [22] . To investigate how WTX regulates these small GTPase members, we first analyzed the interaction of WTX with RhoA, RAC1, and CDC42 by immunoprecipitation (IP), results shown that WTX interacted with CDC42 but not with RhoA or RAC1 in both SW620 and SW480 cells (Fig. 2b and Supplementary Fig. 3b ). Immunofluorescence (IF) staining also shown that WTX and CDC42 co-localized in CRC cells (Fig. 2c ). These data shown that CDC42 might play a critical role in WTX-regulated cell migration. It is known that GTP-bound form of CDC42 is the active state of CDC42 which could transit the signal to the downstream cascades [23] , [24] . As one of the Rho family small GTPase members, CDC42 is a molecular switch that controls cell migration by transformation from the inactive GDP-bound state (CDC42 GDP ) to the active GTP-bound state (CDC42 GTP ) and is overexpressed in colorectal cancer [25] . Since we had found that WTX can interact with CDC42, tour next goal is to investigate the effect of WTX on CDC42 expression and activation in colorectal cancer. We first examined the total CDC42 and CDC42 GTP levels in WTX-overexpressing CRC cells and knockdown CRC cells. Compared with the control cells, CDC42 GTP expression level was dramatically decreased in WTX-overexpressing SW620.W and HT29.W cells but increased in WTX knockdown SW480.shW and HCT116.shW cells. However, the total level of CDC42 was not significantly changed according to WTX express level (Fig. 2d ). These data demonstrate that WTX could inhibit CDC42 by preventing its activation in CRC cells. To test if CDC42 was critical to the metastasis suppressor function of WTX, the suppressed CDC42 GTP levels by WTX was rescued by CDC42 overexpression in SW620.W cells (Fig. 2e ) or the increased CDC42 GTP levels by WTX loss was reversed by CDC42 knockdown in SW480.shW cells (Fig. 2f ). The decreased migration ability of SW620.W cell was recovered by rescuing CDC42 overexpression in SW620.W.CDC cells (Fig. 2g , Supplementary Fig. 3 c ), and the enhanced migration ability of SW480.shW cells was inhibited by CDC42 knockdown in SW480.shW.shC cells (Fig. 2h , Supplementary Fig. 3d ). To further determine the function of CDC42 and CDC42 GTP in WTX loss regulated CRC progress in vivo, we established the colorectal orthotopic xenograft cancer models in nude mice with WTX overexpression (SW620.W) cells and WTX knockdown (SW480.shW) cells. The expression of CDC42 and CDC42 GTP in the mice colorectal orthotopic xenograft tumors were analyzed by IHC. The results showed that the expressions of total CDC42 were relatively stable, but CDC42 GTP were significantly decreased in SW620.W tumor group compared to the SW620.veh control tumor group ( p < 0.05), While CDC42 GTP was increased in SW480.shW tumor group compared to SW480.SCR tumor (only one tumor grew out of five mice, no statistics) (Fig. 2i, j , Supplement Fig. 3e). The mice colorectal orthotopic xenograft tumors models also confirmed that knockdown CDC42 could reverse the WTX-loss related tumor formation and metastasis in vivo (Supplement Figure 4a, b). Those data showed that the activation of CDC42 is critical to WTX-loss induced CRC cells migration and metastasis. 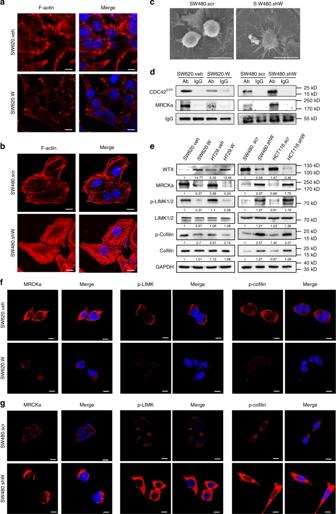Fig. 4 WTX stabilizes F-actin through inhibiting the CDC42 signaling pathway.aIF staining analyzes the expression and location of F-actin in control and WTX-overexpressing cells.bIF staining analyzes the expression and location of F-actin in control and WTX knockdown cells.cScanning Electron Microscopy (SEM) analyzes the cell morphology in indicated cells.dCO-IP analyzes the interactions between MRCKα and CDC42GTPin indicated cells.eIB analyzes the CDC42 pathway proteins in indicated cells.f,gIF staining analyzes the expression and location of MRCKa, p-LIMK1/2, and p-Cofilin in control, WTX overexpression (f) and knockdown (g) cells. Scale bars, 10 μm WTX inhibits CDC42 activation by stabilizing RhoGDIα-CDC42 banding Rho GDP-dissociation inhibitors (RhoGDIs) are important modulators of small GTPases [26] , which switches the small GTPase proteins from active (GTP-loaded) to inactive (GDP-loaded) states. In the inactive state, the protein is stabilized via formation of a complex with the RhoGDIs via the specific binding site of RhoGDIs; in the active state, the protein dissociated with RhoGDIs and formed as GTP-loaded state [27] . Our study confirmed that CDC42 GTP levels in SW620 cells increases after knocking-down RhoGDIa which suggest that the activity of CDC42 was inhibited by RhoGDIa (Fig. 3a ). However, the relationship between WTX and RhoGDIα and the regulatory role of WTX in the RhoGDIα-CDC42 complex forming were still unknown. Fig. 3 WTX inhibits the activation of CDC42 through stabilizing the RhoGDIα-CDC42 binding. a IB analyzes the expression changing of CDC42 GTP in the indicated cells. b CO-IP analyzes the interaction between WTX and RhoGDIa in SW620.W cells. c CO-IP analyzes the interactions between RhoGDIa and CDC42 in the indicated cells. d IB analyzes RhoGDIa and CDC42 expression changes in the indicated cells. e IB analyzes WTX, RhoGDIa and CDC42 expression changes in indicated cells; CO-IP analyzes the interactions between WTX and RhoGDIa, or WTX and CDC42 in indicated cells. f IB analyzes of WTX, RhoGDIa and CDC42 GTP expression changes in indicated cells. g IF staining analyzes the colocation of WTX and RhoGDIa in WTX overexpression cells. Scale bars, 10 μm. h IF staining analyzes the colocation of RhoGDIa and CDC42 in WTX overexpression cells. Scale bars, 10 μm Full size image To investigated the relationship of WTX with RhoGDIα and CDC42, co-IP was performed and confirmed our hypothesis that there was an interaction between WTX and RhoGDIα (Fig. 3b ). CDC42 was stably bond to WTX in parental, WTX knocked down, and overexpressed cells (SW480.shW and SW620.W), but the binding of CDC42 with RhoGDIα was decreased as WTX knocking-down, in contrast, the binding increased as WTX overexpression (Fig. 3c ). We found that CDC42 and RhoGDIα expression level had not changed in WTX-modified cells compared to parental cells (Fig. 3d ). However, CDC42 GTP level was negatively regulated by WTX (Fig. 2d ). WTX expression level did not changed when knocking-down RhoGDIα or CDC42, and it could bind to both RhoGDIα and CDC42 (Fig. 3e ). The results suggested that WTX is the upstream protein and form complex with both RhoGDIα and CDC42, thus regulate CDC42 activity through RhoGDIα. Knocking-down RhoGDIα in either WTX high expression or low expression cells can upregulate CDC42 GTP level (Fig. 3f ), confirming that RhoGDIα was the key mediator to WTX-inhibited CDC42 GTP . Further IF staining demonstrated that WTX has colocation with RhoGDIα (Fig. 3g ) and CDC42 (Fig. 3h ). To uncover whether WNT/β-catenin took effect on WTX/CDC42 signaling axis, β-catenin was knocked down and found that it had not altered the expression of WTX/CDC42 signaling axis downstream molecules like RhoGDIa, CDC42 and the activation of CDC42 (Supplementary Fig. 4c, d ). These data suggest that, by binding to RhoGDIα, WTX formed a complex with RhoGDIα and CDC42, which kept CDC42 inactive, and inhibited it to transform into CDC42 GTP type and therefore prevented the cell migration. Once WTX was lost in tumor cells, the cells will obtain the migration ability and developed into metastasis. This WTX/CDC42 signaling axis was independent of WNT pathway. WTX loss promotes cell migration by causing F-actin polymerization To understand the cell migration mechanism which started by the WTX loss promoted transform of CDC42 GTP , the downstream target needed to be revealed. It is known that CDC42 GTP plays important roles in regulating cell cytoskeleton stability and promoting cell migration and metastasis [15] . Hence, the effect of WTX on cytoskeletal F-actin was examined in both WTX-modified and parental CRC cells by IF staining. The results showed that there were clear plasma membrane blebs and pseudopodia observed in SW620.veh cells. However, the plasma membrane blebs were significantly decreased in size with weaker and shorter pseudopodia (microspikes) in SW620.W cells (Fig. 4a ). Compared with the thin, scanty and short F-actin filaments present in SW480.SCR cells, the F-actin filaments were aggregated into thick, long and parallel F-actin filaments in the plasma and generated clearly polarity in SW480.shW cells (Fig. 4b ). Scanning electron microscopy (SEM) shown that SW480.shW cells exhibited significantly elongated and enlarged pseudopodia, but there were just the few short pseudopodia present in SW480.SCR cells (Fig. 4c ). It demonstrated that WTX loss stimulates F-actin remodeling and polymerization, suggested that it might relate to the abbrent activity of CDC42. In another words, WTX prevented cell migration through inhibition CDC42 GTP to stabilizing F-actin. Fig. 4 WTX stabilizes F-actin through inhibiting the CDC42 signaling pathway. a IF staining analyzes the expression and location of F-actin in control and WTX-overexpressing cells. b IF staining analyzes the expression and location of F-actin in control and WTX knockdown cells. c Scanning Electron Microscopy (SEM) analyzes the cell morphology in indicated cells. d CO-IP analyzes the interactions between MRCKα and CDC42 GTP in indicated cells. e IB analyzes the CDC42 pathway proteins in indicated cells. f , g IF staining analyzes the expression and location of MRCKa, p-LIMK1/2, and p-Cofilin in control, WTX overexpression ( f ) and knockdown ( g ) cells. Scale bars, 10 μm Full size image WTX stabilizes F-actin through inhibiting CDC42 signaling pathway CDC42 downstream signaling cascades MRCKa, LIMK1/2 and Cofilin are involved in the F-actin cytoskeleton remodeling and polymerization pathway [28] . IP experiments were performed to analyze CDC42 downstream proteins and verified that CDC42 GTP could interact with MRCKa, and their interaction was negatively regulated by WTX (Fig. 4d ). Imunoblotting (IB) analysis of the expression levels of CDC42 downstream proteins revealed that, compare with the control cells, CDC42 GTP (Fig. 2d ), MRCKa, p-LIMK1/2, and p-Cofilin were decreased in SW620.W and HT29.W cells but increased in SW480.shW and HCT116.shW cells (Fig. 4e ). There were no significant differences in total CDC42 (Fig. 2d ), LIMK1/2, and Cofilin levels (Fig. 4e ). IF staining also shown that the levels of MRCKa, p-LIMK1/2, and p-Cofilin were reduced in SW620.W cells but increased in SW480.shW cells compared to parental cells (Fig. 4f, g ). These analyzes demonstrated that WTX inhibits the activation of the CDC42, MRCKa, LIMK1/2, and Cofilin signaling pathway, which leads to F-actin stabilization by maintaining cytoskeleton stabilization and blocking the formation of cell filopodia, thus restricts the cell migration. Aberrant miR-20a/106a upregulation leads to WTX loss and CRC progress This study showed that both the protein and mRNA level of WTX were significantly downregulated in CRC patients (Fig. 1a, d ). In addition, WTX mutation was found in only 1 [12] to 10% in CRC [13] . It suggests that there are some other mechanisms that are responsible for WTX loss in CRC patients. It is known that miRNAs regulate their targets by triggering mRNA degradation or translational repression. To explore the mechanism drives WTX loss, we performed miRNAs expression profiling using miRNA arrays in paired cancer and normal colorectal mucosa samples from five CRC patients who has WTX loss in cancer and WTX high in normal colorectal mucosa. Compared with normal tissues, 20 upregulated and 18 downregulated miRNAs with a threefold change were identified in the tumor samples (Fig. 5a ). After we verified the expression level of those miRNAs in human CRC samples, miR-93, miR-20a, and miR-106a were chosen as the candidates. MiR-93, miR-20a, and miR-106a belong to the miR-17 family and share the same core sequences [29] . MiR-93 was tested in 50 pair matched CRC and adjacent mucosa tissue samples showed higher expression in CRC tissues than the matched adjacent colorectal mucosa tissues, but the difference was not significant ( p = 0.1017, Supplementary Fig. 5a ). The miR-20a and miR-106a were further tested in 73 pair matched CRC and adjacent mucosa tissue samples via qRT-PCR. The expressions of miR-20a and miR-106a was significantly higher in CRC samples than in the matched adjacent mucosa tissues ( p < 0.001, Fig. 5b ). The correlation between the expression of miR-20a and WTX were analyzed and confirmed that there was a significant correlation between WTX and miR-20a in CRC patients (Supplementary Fig. 5b ). As miR-20a and miR-106a are more likely to display a similar function in regulating WTX, we then examined both miRNAs in the following analyses. Fig. 5 Aberrant miR-20a/106a upregulation leads to WTX loss in CRC. a MicroRNA expression heatmap of CRC and matched adjacent normal mucosa tissues. b qRT-PCR analyzes miR-20a/106a expression in CRC and matched adjacent normal mucosa tissues. *** p < 0.0001, mean ± SEM. Two-sided paired t -test. c Luciferase activity assay explores WTX 3′-UTR binding with miR-20a or miR-106a in control and SW480 overexpression cells. *** p < 0.0001, mean ± SEM. Two-tailed Student’ s t -test. d IB analyzes WTX expression in indicated cells. e , f Cell proliferation analyzes in indicated cells. * p < 0.05, mean ± SEM. Two-tailed Student’s t -test. g , h Transwell cell migration analyzes in indicated cells. Scale bars, 200 μm. i , j Colony formation analyzes in indicated cell lines. k Gross observation of mice orthotopic CRC tumors and livers. Each arrow pointed a tumor mass. i Quantitative analysis of mice orthotopic CRC tumors in control and miR-20a/106a inhibit SW620 cells. * p < 0.05, mean ± SEM, n = 6. Two-tailed Student’s t -test Full size image To determine if miR-20a and miR-106a indeed binding to WTX gene, their binding sites on WTX gene were predicated by bioinformatics analysis (Supplementary Table 5 ). The actual bindings of miR-20a and miR-106a to the wide type miR-20a/106a binding area on the WTX-3′UTR were confirmed by luciferase assay in SW480 (Fig. 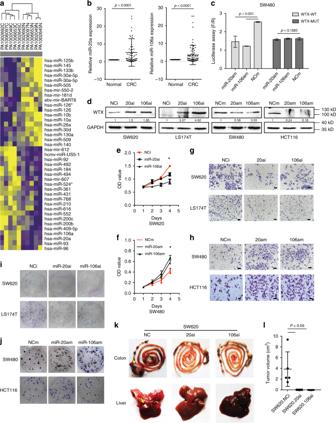Fig. 5 Aberrant miR-20a/106a upregulation leads to WTX loss in CRC.aMicroRNA expression heatmap of CRC and matched adjacent normal mucosa tissues.bqRT-PCR analyzes miR-20a/106a expression in CRC and matched adjacent normal mucosa tissues. ***p< 0.0001, mean ± SEM. Two-sided pairedt-test.cLuciferase activity assay explores WTX 3′-UTR binding with miR-20a or miR-106a in control and SW480 overexpression cells. ***p< 0.0001, mean ± SEM. Two-tailed Student’ st-test.dIB analyzes WTX expression in indicated cells.e,fCell proliferation analyzes in indicated cells. *p< 0.05, mean ± SEM. Two-tailed Student’st-test.g,hTranswell cell migration analyzes in indicated cells. Scale bars, 200 μm.i,jColony formation analyzes in indicated cell lines.kGross observation of mice orthotopic CRC tumors and livers. Each arrow pointed a tumor mass.iQuantitative analysis of mice orthotopic CRC tumors in control and miR-20a/106a inhibit SW620 cells. *p< 0.05, mean ± SEM,n= 6. Two-tailed Student’st-test 5c ), SW620, HCT116, and HEK293A cells (Supplementary Fig. 5 c– e ), with mutated WTX-3′UTR as control. The binding area sequences were verified by BLAST analysis (Supplementary Fig. 5 f, g). These data confirmed that miR-20a and miR-106a could directly bind WTX and are potential regulators of WTX in CRC cells. To farther analyze the biological function of miR-20a/106a and its relationship with WTX, the endogenous expression levels of miR-20a/106a were determined via qRT-PCR in 6 CRC cell lines (SW480, SW620, HCT116, Lovo, LS174T, and HT29) (Supplementary Fig. 5h ). According to the miR-20a/106a qRT-PCR and WTX expression (Fig. 1e ) data, SW620 and LS174T CRC cell lines, which exhibit high miR-20a/106a and low WTX, were selected for establishing miR-20a/106a knocked down cell lines (SW620.20ai/106ai and LS174T.20ai/106ai). SW480 and HCT116 cell lines, which exhibit relatively low miR-20a/106a and high WTX, were selected for establishing miR-20a/106a-overexpressing subclone cell lines (SW480.20am/106am and HCT116.20am/106am) (Supplementary Fig. 6 a, b ). The biological function of miR-20a/106a and their regulation on the expression of WTX were analyzed. Compared with parental cells, WTX expression was significantly increased in SW620.20ai/106ai and LS174T.20ai/106ai cells but reduced in SW480.20am/106am and HCT116.20am/106am cells (Fig. 5d ). Downregulation of both miR-20a and miR-106a could significantly inhibit CRC cell proliferation (Fig. 5e , Supplementary Fig. 6c ), migration (Fig. 5g , Supplementary Fig. 6e, f, i , j), and colony formation (Fig. 5i , Supplementary Fig. 6m, n). Overexpressed miR-20a or miR-106a could enhance CRC cell proliferation (Fig. 5f , Supplementary Fig. 5d ), migration (Fig. 5h , Supplementary Fig. 5 g, h, k, l ), and colony formation (Fig. 5j , Supplementary Fig. 5o, p ). The in vivo subcutaneous mouse model with miR20a and miR106a mimic tumor (Supplementary Fig. 6q, r) confirmed that miR-20a/106a promoted CRC tumor growth. Moreover, the in vivo orthotopic xenograft tumor model shown that the tumor growth and liver metastasis abilities was significantly inhibited when miR-20a/106a expression were reduced (0/6, Fig. 5 k, l, Supplementary Table 6 ). These in vitro and in vivo data demonstrated that miR-20a/106a overexpressing leads to aberrant WTX loss, CRC cell proliferation, and metastasis. 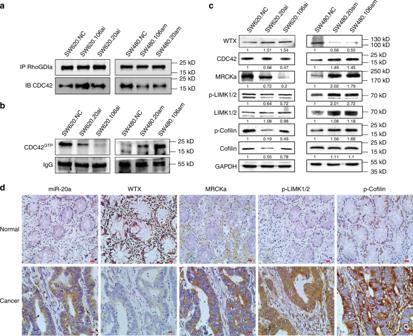Fig. 6 Inhibiting miR-20a/106a rescued the expression of WTX and blocked CDC42 pathway and CRC progression.aCO-IP analyzes RhoGDIa binding with CDC42 in indicated cells.bIB analyzes CDC42GTPexpression in indicated cells.cIB analyzes the expressions of WTX-CDC42-MRCKa-LIMK1/2-Cofilin axis in indicated cells.dISH staining of miR-20a and IHC staining of WTX, MRCKa, p-LIMK1/2, and p-Cofilin expression in CRC and matched colorectal mucosa samples. Scale bars, 20 μm MiR-20a/106a regulated, CRC progression through WTX-CDC42 pathway Since miR20a and miR106a negatively regulated WTX expression (Fig. 5d , and Supplementary Fig. 6a, b ), we next tested if miR-20a/106a could affect the stability of WTX/RhoGDIα/CDC42 complex, the CDC42 downstream signaling pathway activity and CRC progression. Firstly, IP western analysis shown that the binding of CDC42 to RhoGDIα was also negatively regulate by miR-20a/106a (Fig. 6a ), combined with miR-20a/106a negatively regulate WTX expression (Figs. 5d and 6c ), those findings confirmed that miR-20a/106a regulates RhoGDIα/CDC42 complex formation through inhibiting WTX expression to promote CDC42 GTP transformation. Consequently, the WTX/RhoGDIα/CDC42 downstream pathway, MRCKa, P-LIMK, and P-Cofilin, were also activitied in CRC cells (Fig. 6c ). These results further suggested that miR-20a/106a regulates the WTX/RhoGDIα/CDC42 pathway through repressing WTX and blocking RhoGDIα bond to CDC42, which subsequently activated the CDC42 pathway in CRC cells. Fig. 6 Inhibiting miR-20a/106a rescued the expression of WTX and blocked CDC42 pathway and CRC progression. a CO-IP analyzes RhoGDIa binding with CDC42 in indicated cells. b IB analyzes CDC42 GTP expression in indicated cells. c IB analyzes the expressions of WTX-CDC42-MRCKa-LIMK1/2-Cofilin axis in indicated cells. d ISH staining of miR-20a and IHC staining of WTX, MRCKa, p-LIMK1/2, and p-Cofilin expression in CRC and matched colorectal mucosa samples. Scale bars, 20 μm Full size image To further investigate the clinical relevance of the miR-20a/106a/WTX/RhoGDIα/CDC42 signaling pathway in CRC progression, the 3D invasion experiments had performed and shown that inhibition of miR-20a/miR-106a could inhibit CRC cell 3D sphere growth and invasion, while overexpression of miR-20a/miR-106a could improve CRC cell 3D sphere growth and invasion (Supplementary Figure 7a, b, p < 0.001). The key components of this signaling cascades were also examined by ISH or IHC staining in human CRC patients and matched normal colorectal mucosa tissues. 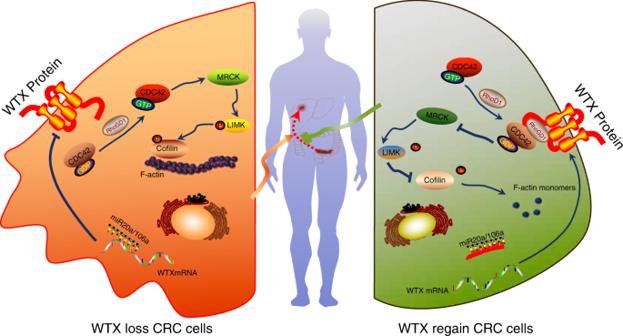Fig. 7 The mechanism of Mir20a/106a-WTX axis regulates RhoGDI/CDC42 signaling and their function in CRC progression. In CRC cell, the aberrant high miR-20a/106a inhibits WTX expression. Without WTX, RhoGDIα could not form the stable RhoGDIα/CDC42 complex, subsequently the CDC42GDPdissociats from RhoGDIα and transforms to CDC42GTPand becomes active. Then CDC42GTPactivates the downstream MRCKa-LIMK1/2-Cofilin pathway, which results in F-actin remodeling, increased cell proliferation, polarity, and migration ability, finally promots CRC progression and liver metastasis. To block miR-20a/106a could recover WTX expression. The regained WTX promots RhoGDIα/CDC42 complex formation and keeps it stability, so that CDC42 stays inactivity by keeping in the CDC42GDPtype which inhibits MRCKa-LIMK1/2-Cofilin pathway, thus prevents CRC progression and liver metastasis (all the images in the figure are created by Q.-l. Z, polished by C. L and H. W.) Compared to mucosa tissues, CRC tissues has significantly higher expression of miR-20a, MRCKa, p-LIMK1/2, and p-Cofilin, and significantly lower expression of WTX (Fig. 6d and Supplementary Fig. 7c–f ). Together, these results confirmed that miR-20a/106a inhibits WTX expression and subsequently activated the CDC42 pathway to catalyze the CRC progression and liver metastasis. 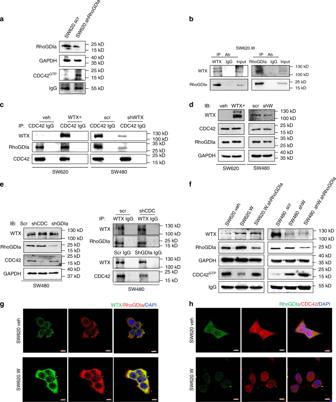It is well-known that WTX functions as a tumor suppressor in Wilms tumor, and its classical role in Wnt/β-catenin signaling pathway. However, the role of WTX in the other types of cancers is not illustrated and the functions of WTX are not well explored. In this study, we discovered that WTX expression negatively correlated with metastasis, stages, and poor survival in human CRC patients. Further in vivo and in vitro analyses validated that WTX acts as a tumor suppressor gene in CRC cell lines by preventing cell proliferation, cell migration, tumor formation, and liver metastasis. Fig. 3 WTX inhibits the activation of CDC42 through stabilizing the RhoGDIα-CDC42 binding.aIB analyzes the expression changing of CDC42GTPin the indicated cells.bCO-IP analyzes the interaction between WTX and RhoGDIa in SW620.W cells.cCO-IP analyzes the interactions between RhoGDIa and CDC42 in the indicated cells.dIB analyzes RhoGDIa and CDC42 expression changes in the indicated cells.eIB analyzes WTX, RhoGDIa and CDC42 expression changes in indicated cells; CO-IP analyzes the interactions between WTX and RhoGDIa, or WTX and CDC42 in indicated cells.fIB analyzes of WTX, RhoGDIa and CDC42GTPexpression changes in indicated cells.gIF staining analyzes the colocation of WTX and RhoGDIa in WTX overexpression cells. Scale bars, 10 μm.hIF staining analyzes the colocation of RhoGDIa and CDC42 in WTX overexpression cells. Scale bars, 10 μm Data presented above suggest that WTX loss plays an important role in CRC progress, especially in liver metastasis. Since liver metastasis is the leading cause of CRC patient death, understanding the mechanisms underlying WTX loss driven liver metastasis has potential to vastly improving the survival rate of CRC patients by preventing CRC progression. CDC42 has been characterized for regulating various cellular responses including cellular transformation, cell invasion, cell polarity, and migration [30] . Similar to most Ras-related proteins, CDC42 GTPases act as switches exchanging between inactive GDP-bound form (CDC42 GDP ) and active GTP-bound form (CDC42 GTP ) [31] . Our study demonstrate WTX physically interacts with CDC42 but not RhoA or Rac1 in CRC cells, and WTX loss activates CDC42 and its downstream signaling pathway. CDC42 promotes the invasion and migration of many human cancers, including CRC [32] , lung cancer [33] , breast cancer [34] , esophageal cancer [35] , [36] , gastric cancer [37] , renal cell cancer [38] , cervical cancer [17] , etc. And high CDC42 expression has been reported to correlate with CRC development, CDC42 can be used as a biomarker and therapeutic target of CRC [25] , [39] . Thus, targeting CDC42 might inhibit the WTX loss driven CRC progression and metastasis. To uncover the mechanism of WTX regulating CDC42, the relationship of WTX with Rho GDP-dissociation inhibitor 1 (RhoGDIα, RhoGDI1) was analyzed. RhoGDIα is one of the regulatory proteins required for the GDP/GTP exchange reaction, which inhibits CDC42 activation by forming a tight 1:1 cytosolic complex [40] , [41] and retaining it in the inactive cytosolic pool (CDC42 GDP state) [42] . Thus, RhoGDIα plays an essential role in CDC42-mediated cellular transformation [43] . Here, we found that WTX inhibits CDC42 activation through binding to RhoGDIα and then stabilizing the complex formation of RhoGDIα and CDC42. Thereby, RhoGDIα retains CDC42 in the inactive form and inhibits its functions. This study identified an unknown mechanism that loss of WTX promotes CRC cell proliferation, viability, and metastasis through untying RhoGDIα, then disrupting the interaction of RhoGDIα and CDC42, cause the increasing of CDC42 GTP levels. CDC42 participates in steps of cell proliferation and migration regulation, it is essential for actin-based motility by regulating actin reorganization [44] , [45] . This study demonstrates that WTX inhibits F-actin remodeling and polymerization, which blocks cytoskeletal reorganization and the development of polarity in CRC cells. In addition, WTX loss promotes CDC42 GDP transition to CDC42 GTP and then activates downstream of MRCKa, p-LIMK1/2, and p-Cofilin, and initiated F-actin remodeling, thus enhancing CRC cell polarity and migration. Mutation is an important factor responsible for tumor suppressor genes silencing. Mutation of the WTX gene has been widely reported in Wilms tumors [1] , [8] , [46] , [47] , [48] , leukemia [49] , CRC [12] , [13] , and alimentary carcinomas [11] , [12] . However, high diversity of mutation rates of WTX were observed in Wilms tumors and alimentary carcinomas, suggesting that WTX gene mutation is not the pivotal cause of WTX silencing. miRNA regulation is another important factor in tumor suppressor gene silencing [50] , [51] . To find out the reasons to drive WTX loss in CRC, microRNA array analyses were used and screened out miR-20a/106a as candidates to regulate WTX in this study. Mir-20a/106a has been reported to promote multiple types of cancer growth and metastasis through different mechanism. For example, miR-20a promotes cervical cancer proliferation and metastasis in vitro and in vivo [PMID: 25803820], and miR-20a triggers metastasis of gallbladder carcinoma [PMID: 23665284]. Oncogenic miR-20a and miR-106a enhance the invasiveness of human glioma stem cells by directly targeting TIMP-2 [PMID: 24704830]. MiR-20a induces cell radioresistance by activating the PTEN/PI3K/Akt signaling pathway in Hepatocellular Carcinoma [PMID: 26031366]. So, the relationship of miR-20a/106a with WTX were analyze in human samples, the result demonstrated that aberrant high expression of miR-20a/106a correlate with WTX loss in CRC patients. Thus, it revealed the probably reason of WTX loss in CRC. Further studies revealed WTX is a target of miR-20a/106a in CRC cells, and miR-20a/106a negatively regulates WTX/RhoGDIα/CDC42-MRCKa-LIMK1/2-Cofilin pathway by preventing WTX expression thus promoting CRC liver metastasis. Previous studies have found that miR-20a/106a overexpressed in CRC is correlated with aggressive biological behaviors, including promotion of the cell cycle [52] , drug resistance [53] and RB tumor suppressor gene inhibition [54] , therefore our study uncovered the function and mechanism of miR-20a/106a in CRC, and as miR-20a/106a drive WTX loss induced CRC cells to gain the migration ability, we can predicate that inhibiting miR-20a/miR-106a might provide an intriguing target for CRC treatment. Overall, our study revealed a metastatic suppressor functions of WTX in CRC progression and liver metastasis and identified a new mechanism accounts for WTX loss. MiR-20a/106a inhibits WTX expression, blocks RhoGDIα/CDC42 complex formation, subsequently promotes CDC42 GDP dissociation from RhoGDIα and transformation into CDC42 GTP , thus activating the downstream pathway which results in F-actin remodeling, increased cell proliferation, polarity, and migration ability, and finally leads to catalyzing CRC progression and liver metastasis (Fig. 7 ). This study also suggests that targeting miR-20a/106a or CDC42-MRCKa-LIMK1/2-Cofilin pathway could be developed into a therapy to treat CRC progression and metastasis. Fig. 7 The mechanism of Mir20a/106a-WTX axis regulates RhoGDI/CDC42 signaling and their function in CRC progression. In CRC cell, the aberrant high miR-20a/106a inhibits WTX expression. Without WTX, RhoGDIα could not form the stable RhoGDIα/CDC42 complex, subsequently the CDC42 GDP dissociats from RhoGDIα and transforms to CDC42 GTP and becomes active. Then CDC42 GTP activates the downstream MRCKa-LIMK1/2-Cofilin pathway, which results in F-actin remodeling, increased cell proliferation, polarity, and migration ability, finally promots CRC progression and liver metastasis. To block miR-20a/106a could recover WTX expression. The regained WTX promots RhoGDIα/CDC42 complex formation and keeps it stability, so that CDC42 stays inactivity by keeping in the CDC42 GDP type which inhibits MRCKa-LIMK1/2-Cofilin pathway, thus prevents CRC progression and liver metastasis (all the images in the figure are created by Q.-l. Z, polished by C. L and H. W.) Full size image Tissue specimens One hundred and seventeen matched human CRC and normal tissue specimens were collected at Nanfang Hospital, Southern Medical University between 2008 and 2011. Patient samples were collected and processed in compliance with protocol approved by Southern Medical University (Guangzhou, China) Institutional Review Board. None of these patients received chemotherapy or radiation therapy before surgery. We used archived samples. At the time of tissue collection, informed consent was obtained from all patients. Reagents and tissue samples Clean-Blot IP detection reagent (HRP) (21230) for clean IP detection was purchased from Thermo Scientific Company. The primers sequences for WTX gene CDS and qRT-PCR were listed in Supplementary Tables 2 and 3 . GeneChem (ShangHai, China) synthesized the siRNAs, the sequences shown in Supplementary Table 4 . Primary antibodies information shows in Supplementary Table 7 . Secondary antibodies conjugated to Alexa 488 or Alexa 594 for immunofluorescence staining and conjugated to HRP for Immunoblotting were purchased from ZSGB-BIO (Guangzhou, China), Rhodamine Phalloidin was purchased from Cytoskeleton Inc (USA). Tissue samples were obtained from patients who had undergone routine surgery at Nanfang Hospital, Southern Medical University, China, between 2005 and 2015. The informed consent was obtained from all human participants. Immunohistochemistry (IHC) The paraffin-embedded sections were stepwise dewaxed from xylene, gradient ethanol to water, and performed immunohistochemical staining as protocol. IHC staining was performed with heat-induced antigen retrieval, followed by incubating in primary antibodies overnight at 4 ℃, secondary antibody (EnVision/HRP kit, DAKO) 30 min at RT (room temperature) and substrate-chromogen solution (DAB detection kit, DAKO) 5–10 min at RT, with hematoxylin counterstain for 10 s. Among each step, washing the slides in PBS three times for 5 min. Normal kidneys were used as positive controls; normal serum in place of the primary antibody as an isotype negative control, and the slides without added primary antibody were used as negative controls. The results were scored as previously described and scored as a sum of the staining intensity and percentage of positive tumor cells. Briefly, the staining intensity scaled with 0–3. Percentage of positive cells staining was scored as 0–4. The final staining was summed by intensity and percentage as 0–12. And then adapted to 4-point IRS: 0–1 (−), 2–3 (+), 4–8 (+ +), and 9–12 as (+ + +). 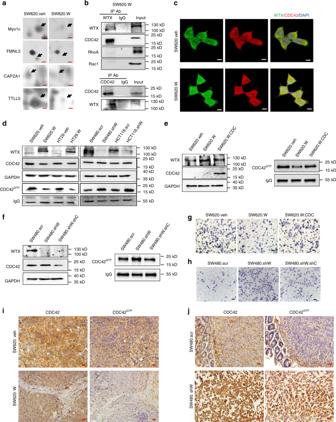Finally, we set “+“ as WTX expression cut off point: − as negative;+ ~ + + + as positive [4] . The clinical pathologic meanings of the IHC data were analyzed by Chi-square analysis. IHC staining and statistics were performed in a blind manner. RNA extraction and quantity real-time PCR (qRT-PCR) Total mRNA was extracted from human CRC and matched adjacent normal mucosa tissues or six CRC cell lines with RNAiso-Plus (TAKARA, DaLian, China). Single-stranded cDNA was then synthesized from 1 μg extracted mRNA by using the qRT-PCR cDNA synthesis kit (TAKARA, DaLian, China) according to the manufacturer’s instructions. Fig. 2 Inhibition of CDC42 activity prevents WTX loss induced CRC cell migration.a2-DGE searches the difference protein expression dots between SW620.veh and SW620.W cells. Scale bars, 500 μm.bCO-IP analyzes the interaction of WTX and Small GTPases family members in SW620.W cells.cIF staining analyzes the colocation of WTX and CDC42 in SW620.veh and SW620.W cells. Scale bars, 10 μm.dIB analyzes the expression level of CDC42 and CDC42GTPin indicated cell lines.e,fIB analyzes the expressions of WTX, CDC42 and CDC42GTPin indicated cells.g,hTranswell experiments analyze the migration ability in indicated cells. Scale bars, 200 μm.i,jIHC staining analyzes the expressions of CDC42 and CDC42GTPin CRC orthotopic tumors. Scale bars, 20 μm Real-time PCR was performed by the Applied Biosystems 7500 Sequence Detection system with the iQ™ SYBR green supermix (Bio-Rad Laboratories, Hercules, CA, USA) containing 1/10 of total volume cDNA and 10 nmol of each pair of the sense and anti-sense primers (sequences shown in Supplementary Table 2 ). The cycling conditions were: 95 °C 5 min for 1 cycle; 95 °C 5 s, 60 °C 30 s, and 72 °C 34 s for 40 cycles followed by the melting curve stage. The relative expression of WTX gene was evaluated based on the threshold cycle (Ct), and calculated as 2 −ΔΔCT . All of the samples get three independent experiments with four technical replicates each day. Cell lines and cell culture The human CRC cell lines SW620, SW480, HCT116, HT29, LOVO, and LS174T were obtained from the American Type Culture Collection (ATCC), generated, in the Department of Pathology, Nanfang Hospital, and were authenticated and tested for mycoplasma contamination. SW620 derived from metastatic Lymph Node. LOVO derived from metastatic left supraclavicular region. The other cell lines were derived from CRC tissues. All of the cell lines and the modified variants were cultured in RPMI 1640 (BI) full medium with 10% FBS, and the HEK293T cell line was cultured in DMEM (GIBCO) full medium with 10% FBS at 37 °C in a humidified atmosphere of 5% CO 2 . WTX full-length plasmid implication, overexpression, and knockdown The 3408 bp full WTX gene CDS sequence were amplified by using GeneArt® Gene Synthesis technique with EcoRI and BamHI restriction enzyme sites at ends. The primers sequences were listed on Supplementary Table 2 . The WTX gene was cloned into pEGFP-N1 vector (Invitrogen, Shanghai, China) to construct pEGFP-N1-WTX vector and verified by sequence analysis. Then, the pEGFP-N1-WTX vector was transfected into SW620 and HT29 cells to establish the WTX overexpression subclone cell lines. The shRNA of WTX, CDC42, and RhoGDIa were purchased from Origene Company (Beijin, China) and transfected into SW480 and HCT116 cells to establish the WTX knockdown subclone cell lines. Cell proliferation, migration, and colony formation assays Cell counting kit-8 (CCK8) was used for cell proliferation assay, 1 × 10 3 cells were seeded on 96-well plates and cultured for 24 h. Hundred microliters of CCK8 buffer (Dojindo, Japan) was added to each well and incubated for 2 h. The absorbance was measured at 450 nm using Microplate Autoreader (Bio-Rad, Hercules, CA, USA). The experiment was repeated for three times under the same condition. For cell migration assay, 1 × 10 5 cells were seeded onto Transwell chambers (BD Biosciences, SanJose, CA, USA) under the same treatment conditions and incubated for 48–72 h. Cells that had migrated the filter were stained with hematoxylin and counted in five fields per insert for further statistical analysis. For would healing assays, the pretreated sub-line cells were seeded into 6-well plated and scratched with a pipette tip in 24 h, after the clearance of wounded floating cells with PBS, the cells were continuously cultured for another 48 h and took photos in every 6 h. For colony formation assay, cells were seeded on six-well plates in 300 cells/well and cultured 2 weeks until the visualization cell colonies appeared. The colonies were then stained with hematoxylin for 30 min after 30 min of fixation by 4% paraformaldehyde. The colony numbers, defined as >50 cells/colony, were then counted for further statistical analysis. The error bars represent mean ± SEM from three independent experiments. Cell 3D culture Single cells were seeded in 24-well chamber culture slides (BD Falcon) on a bed of LDEV-free MatriGel (Corning) in RPMI supplemented with 10% FBS and 5% MatriGel. Two days after seeding cells, media was replaced in all conditions. Three days after seeding cells, pictures were taken on microscope every 3 days. Sphere area was quantified using ImageJ on 20–30 colonies per replicate. Two-dimensional page electrophoresis (2-DGE) and mass spectrometric analysis Protein extraction was performed from the stable WTX overexpression cells (SW620.W) and control cells (SW620.veh). For 2-DGE analysis, SW620.W or SW620.veh cell protein was loaded onto the immobilized pH gradient (IPG) Drystrip (pH 3–10, 24 cm, GE Healthcare, Piscataway NJ, USA). The strips were subsequently placed on the top of vertical 12.5% SDS-polyacrylamide self-cast gels and subjected to electrophoresis using an Ettan™ DALT system (GE Healthcare). After being stained by Colloidal Coomassie Blue G-250, the gels of SW620.W and SW620.veh cells were scanned and analyzed by using PD Quest software (Version 7.0, Bio-Rad). The interested DPDs were selected and identified by Mass spectrometric analysis. Immunoprecipitation and immunoblotting For immunoprecipitation, cellular lysates were incubated with antibody overnight, followed by incubating with protein A/G-sepharose beads (Santa Cruz Biotechnology) for 4 h; 2500 × g centrifugation and three times washing with ice-cold lysis buffer. The immunoprecipitated proteins were eluted by denaturation Laemmli buffer at 95 ℃ for 5 min; separated by SDS-PAGE gel, transferred to a PVDF membrane (Pierce), blocked with 5% nonfat milk and incubating with primary antibodies, then secondary antibodies. The protein was finally visualized using enhanced chemiluminescence detection system (Amersham Biosciences Europe, Freiberg, Germany) according to the manufacturer’s instructions. CDC42 activation assay Cellular protein lysates were incubated with active antibody of CDC42 who specifically recognizes CDC42 GTP overnight at 4 ℃. Then the lysate-active antibody complex was incubated with protein A/G-sepharose beads at 4 °C for 1 h with gentle agitation. After centrifugal collection, washing and resuspending with protein loading buffer, the lysate-active antibody complex was eluted from sepharose beads by boiling 5 min; followed by standard Immunoblotting to quantity CDC42 GTP amount in procedures as Cdc42 Activation Assay Kit protocol (ab173238, Abcam, Cambridge, UK). Immunofluorescence Grouped cell lines were seeded on confocal disks and cultured in full medium for 12 h. Then washed and fixed them in 4% formaldehyde for 30 min, permeabilization with 0.2% Triton-100 for 15 min, and incubated with primary antibody overnight and Alexa488/594 conjugated secondary antibody or rhodamine phalloidin (Cytoskeleton Inc., Denver, USA) for 1 h and followed by DAPI counterstaining for 10 min. Then observed by the Olympus confocal fluorescence microscope (Fluoview FV1000). Scanning electron microscopy (SEM) Cells were seeded on 12 × 12 mm pre-cleaned coverslips and cultured in 24-well plates for 36 h. Then followed by being washed in PBS for three times and fixed in 2.5% glutaraldehyde for 4 h at RT, rewashed in PBS for two times, dehydrated by using graded ethanol at 4 ℃, soaked in 100% acetonum for 20 min, and 100% isoamyl acetate 15 min and propylene epoxide for 20 min at 45 ℃, the coverslips were then vacuumed and spray coated with metal foil and put under the Scanning Electron Microscopy for further observation. MiRNA array Total RNA of CRC and matched colorectal mucosa tissue was extracted by using the RNeasy Kit (Qiagen) and labeled by Hy3 with miRCURY LNA miRNA Power Labeling Kit (Exqion, USA), using Human Lung fibroblast cell lines (HLF) as sample controls which being labeled by Hy5. MiRNA microarrays (CCDTM-miRNA850-V4p1.4) were provided by Infectious Disease and Immunogenetics section, Department of Transfusion Medicine, Clinical Center, National Institutes of Health, USA [55] . After incubating the RNA samples in miRNA arrays at room temperature overnight, images were then collected with LuxScan TM 10 K microarray Scanner (Bioss, Germany) and processed with BRB-ArrayTools(USA). Statistics and plotting were conducted using the software R v2.15.3 with the Bioconductor packages [56] . Detailed data analyzed with Cluster and Treeview software (EisenLab). Dual-luciferase reporter system analysis WTX gene 3′UTR fragment, which covered miR-20a/106a binding site, was amplified from genomic DNA by PCR. The primers sequences were listed in Extended Supplementary Table 2 . The specifically mutated WTX gene 3′UTR fragment was obtained by using QuickChange site-directed mutagenesis kit (TOYOBO). They were subcloned into the pGL3-control vector (Promega) to construct pGL3-WTX-3′UTR-WT or pGL3-WTX-3′UTR-Mut vectors, respectively. Co-transfect the vectors and miR-20a or miR-106a to SW480, HEK293A or HCT116 cells, harvest the cells in 48 h and analyzed for luciferase activity using Dual-luciferase reporter assay system (Promega) and PerkinElmer detection system (EnSpire 2300 multilabel reader) according to the manufacturer’s instructions. Three repeat experiments were conducted independently. MiRNA expression and function analysis SW480 and HCT116 cells were selected for transfecting miR-20/106a mimics, SW620 and LS174T cells were selected for transfecting miR-20/106a inhibitors. The cells were seeded in 6-well culture plates overnight and transfected in Opti-MEM medium with miR-20a/106a mimics, inhibitors or control (GenePharma, Shanghai, China) using Lipofectamine 2000 (Invitrogen, Carlsbad, CA, USA) transfecting agent according to the manufacturer’s protocol. Briefly, 10 μl miR-20/106a mimics, inhibitors or controls (100 nM) were diluted with 250 μl serum-free medium and incubated 5 min at RT; at the same time, added 5 μl lipofectamine 2000 in 250 μl serum-free medium and incubated 5 min at RT. Then, mixed and incubated the two complexes for 20 min at RT and added them to the aim cells; tested the miR-20, miR-106a, and WTX expression level by qRT-PCR in 48 h of transfection. The biological function studies of cell proliferation and migration were analyzed by following the above protocol. Animal information All mice were housed under specific pathogen-free (SPF) conditions and all animal models complied with all relevant ethical regulations. The study protocol was approved by the Institute Animal Care and Use Committee of Nanfang Hospital, Southern Medical University. Subcutaneous or orthotopic xenograft colorectal tumor models were established in 4–6-week-old BALB/c athymic nude mice (Animal Center of Southern Medical University, Guangzhou, China). Subcutaneous CRC mouse model The SW480 and SW620 cells were harvested and suspended by fresh PBS to a concentration 1 × 10 6 cells/100 μl. Slowly pull-up 100 μl of cells using an insulin syringe. Pinch the skin, inject the 1 × 10 6 cells slowly and evenly into the pouch, creating a single bubble of cells beneath the skin. Seven days later, the tumor sizes were started to be measured twice a week using a caliper. The subcutaneous tumor volumes were calculated by the formula: V = ( a × b 2 )/2. After 30 days observing, the mice were sacrificed to harvest the tumor for farther analysis and establish the proliferation curve. Orthotopic xenograft colorectal cancer mouse model The SW480 and SW620 cells were prepared and suspended by fresh PBS to a concentration 1 × 10 6 cells/50 μl and aspirated by finer needle. The mice were anesthetized and exposed the cecum by the laparotomy. In briefly, a 0.5~1 cm long small nick in the skin was made, and the abdominal wall musculature was lifted, the abdominal cavity was open, the cecum was isolated and covered by warm saline sterile gauze to keep the cecum moist. Slowly injected a 50 µL volume of cells into the cecal wall. Carefully removed the needle and inspected the injection site to ensure no leakage. Then returned the cecum to the abdominal cavity and closed the abdominal wall and skin. Sixty days later, the mouse was sacrificed and to measure and harvest the orthotopic xenograft colorectal cancer masses for farther study. If the tumor mass was invisible, embedded the full intestine to calculate the maximum tumor size under microscopy. In situ hybridization (ISH) All steps were performed under RNase-free conditions. The miR-20-3p, miR-20-5p probes and ISH kit were purchased from Boster Company (Wuhan, China). The slides were stepwise dewaxed from xylene, gradient ethanol to water, and re-fixed by 4% paraformaldehyde by DEPC-PBS for 10 min. Then they were incubated in 50 µg/ml Proteinase K, prehybridise for 4 h at 60 °C, 1.5 µg/ml probe incubated 18 h at 60 °C in series; following 2 × SSC, 1 × SSC, and 0.1 × SSC strict rinsing; blocking, anti-digoxin biotin, SABC-POD, streptavidin-HRP, DAB substation, and hematoxylin counterstain in sequence to detect the positive signal. Score and statistical analysis The IHC and ISH signaling was scored and analyzed as the previous protocol [57] . Statistical analysis was performed using GraphPad Prism (Prism 5.0; GraphPad Software Inc.) packages. The enumeration data analyzed by using t- test, the measurement data analyzed by using χ 2 test. Survival curves of WTX expression in CRC patients were analyzed using the Kaplan–Meier method and assessed by log-rank testing. p < 0.05 was considered statistically significant. Error bars indicate the standard deviation in all the Figures.